Multi-localization transport behaviour in bulk thermoelectric materials Simultaneously optimizing electrical and thermal transport properties of bulk thermoelectric materials remains a key challenge due to the conflicting combination of material traits. Here, we have explored the electrical and thermal transport features of In-filled CoSb 3 through X-ray absorption fine structure, X-ray photoemission spectra, transport measurement and theoretical calculation. The results provide evidence of three types of coexisting multi-localization transport behaviours in the material; these are heat-carrying phonon-localized resonant scattering, accelerated electron movement and increase in density of states near the Fermi level. The 5 p -orbital hybridization between In and Sb is discovered in the In-filled CoSb 3 compound, which results in a charge transfer from Sb to In and the enhancement of p–d orbital hybridization between Co and Sb. Our work demonstrates that the electrical and thermal properties of filled skutterudite bulk thermoelectric materials can be simultaneously optimized through the three types of coexisting multi-localization transport behaviours in an independent way. Thermoelectric (TE) devices, which can directly convert heat into electricity and vice versa, have attracted considerable attention due to a variety of applications in heating, cooling, power generation and waste heat recovery [1] . Their conversion efficiency depends on the dimensionless figure of merit of TE materials defined as ZT =α 2 σT/κ , where T is the absolute temperature, σ is the electrical conductivity, α is the Seebeck coefficient and κ is the total thermal conductivity ( κ=κ E +κ L , where κ E is the electronic contribution and κ L the lattice contribution). Numerous efforts have been attempted to improve ZT in the past two decades despite a compromise of κ and α with σ in TE materials [2] . To decrease κ L , various approaches used to enhance phonon scattering have taken advantage of nanoinclusion [3] , [4] , [5] , [6] , alloying [7] , rattling filler [8] , quasi-ballistic transport nanoscale interfaces or nanopores [9] , [10] , liquid-like behaviour copper ions [11] and anharmonic phonon coupling [12] . Meanwhile, a series of band structure engineering approaches such as high valley degeneracy [13] , [14] , peierls distortion [15] , electron energy filtering near the Fermi level [16] , [17] , [18] and optimal bandwidth [19] , have been employed to improve the electrical properties. Some important single-localization transport behaviours have been discovered in different TE materials. For example, interface scattering in AgPb m SbTe 2 + m (ref. 4 ) and BiSbTe (ref. 6 ), and localized resonant scattering in filled CoSb 3 (ref. 8 ) have remarkably enhanced phonon scattering and reduced κ L ; band convergence in PbTe 1− x Se x (ref. 13 ) and Mg 2 Si 1− x Sn x (ref. 14 ), charge density wave in In 4 Se 3 (ref. 15 ) and electron resonant state in PbTe (ref. 16 ) have all led to an effective increase in α . These single-localization transport behaviour, however, can only optimize a single physical parameter of electrical or thermal properties. So far, it remains a major challenge to simultaneously increase α and σ while reducing κ , because no material has been found that shows multiple-localization transport behaviour. Filled CoSb 3 have been intensely pursued as an important TE material for intermediate-temperature power generation. The major progress in improving ZT has made through decreasing κ L by filling the icosahedron voids in CoSb 3 with foreign atoms (for example, rare earths, alkali earths or alkali metals) to enhance heat-carrying phonon-localized resonant scattering via filler rattling [8] , [20] , [21] , [22] , [23] , [24] , [25] , [26] , [27] , [28] , [29] . Shi et al . [28] suggested that the electrical properties of multiple-filled CoSb 3 could be optimized by adjusting the total filling fraction of fillers with different charge states. However, the tuning space of electrical properties is limited due to the conflicting relationship among α , n and σ , as expressed in the following formulae: where m * is the carrier effective mass; n , the carrier concentration and μ H , the carrier mobility. Recently, more and more experiments indicate that group III elements (Ga, In and Tl) can remarkably improve ZT of CoSb 3 materials because of an almost perfect combination of low κ L , high σ and large α [30] , [31] , [32] , [33] , [34] , [35] , [36] , [38] . However, it still remains unsettled how the group III elements synergistically adjust the electrical and thermal properties of CoSb 3 . The Tl filler rattling only explains the low κ L of Tl-filled CoSb 3 (refs 30 , 31 ). The dual-site occupancy at both the voids and Sb sites for Ga in CoSb 3 is only responsible for low κ L and n [32] . Up to now, the doping behaviour of the In impurity in CoSb 3 remains an ongoing debate [33] , [34] , [35] , [36] , [38] , [39] , [40] , [41] , [42] . In the following, we have explored the electrical and thermal transport features of In-filled CoSb 3 through X-ray absorption fine structure (XAFS), X-ray photoemission spectra (XPS), transport measurement and theoretical calculation. Our data suggest that there are three types of coexisting multi-localization transport behaviours including heat-carrying phonon-localized resonant scattering, accelerated electron movement and increase in density of states (DOSs) near the Fermi level. Our work demonstrates that the electrical and thermal properties can be independently optimized through the three types of coexisting multi-localization transport behaviours. Filling behaviour of In impurity in CoSb 3 We compare In K -edge X-ray absorption near-edge structure (XANES) experimental spectra of quenched In 0.2 Co 4 Sb 12 (Q 0.2 ) and annealed In x Co 4 Sb 12 ( x =0.1, 0.2 and 0.25) (A x ) with those of InSb and In metal ( Fig. 1 ). The In K -edge XANES spectrum of the In metal has five absorption peaks A 1 , B 1 , C 1 , D 1 and E 1 centred at about 9, 28, 52, 84 and 128 eV, respectively, whereas that of InSb has four absorption peaks A 2 , B 2 , C 2 and D 2 at about 11, 35, 64 and 107 eV, respectively. The In K -edge XANES spectrum of Q 0.2 has four absorption peaks with almost the same positions as those of InSb, indicating the existence of InSb in Q 0.2 . 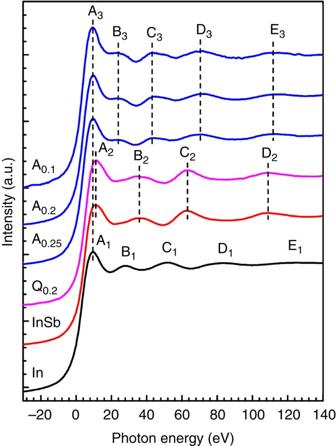Figure 1: The InK-edge XANES experimental spectra. The quenched In0.2Co4Sb12is symbolized with ‘Q0.2’. The annealed InxCo4Sb12(x=0.1, 0.2 and 0.25) is symbolized with ‘Ax’. The InK-edge XANES experimental spectra of InSb and In metals are plotted for comparison. Zero eV corresponds to the threshold of InK-edge (27,940 eV). Figure 1: The In K -edge XANES experimental spectra. The quenched In 0.2 Co 4 Sb 12 is symbolized with ‘Q 0.2 ’. The annealed In x Co 4 Sb 12 ( x =0.1, 0.2 and 0.25) is symbolized with ‘A x ’. The In K -edge XANES experimental spectra of InSb and In metals are plotted for comparison. Zero eV corresponds to the threshold of In K -edge (27,940 eV). Full size image All the In K -edge XANES spectra of the A x samples encompass five absorption peaks A 3 , B 3 , C 3 , D 3 and E 3 with energy near 9, 23, 42, 70 and 113 eV, respectively. The main peak A 3 has the same energy as that of A 1 for the In metal, but is 2 eV lower than that of A 2 for InSb. For the In K -edge XANES spectra, the main peaks A 1 , A 2 and A 3 can be attributed to the 1 s →5 p transition. The energy discrepancy of A 2 and A 3 indicates that the chemical states of the In impurity are different between the A x samples and InSb. It is worth noting that the absorption peaks B 3 , C 3 , D 3 and E 3 of all the A x samples are distinctly different in energy from B 1 , C 1 , D 1 and E 1 for the In metal, and from B 2 , C 2 and D 2 of InSb. Such significant differences undoubtedly show that the In impurities in the A x samples are neither InSb nor the In metal. Accordingly, it is highly plausible that the In impurities have been incoporated in the lattice of CoSb 3 in all annealed samples, well consistent with the X-ray diffraction results (see Supplementary Fig. 1 ). Because of the close electronegativity values among In (1.78), Sb (2.05) and Co (1.88), there exist four possible occupational sites for the In impurities in CoSb 3 , filling the icosahedron voids at the 2 a sites to form In-filled CoSb 3 , substituting for Sb at the 24 g sites in the disordered Sb 2 Co 2 tetrahedron to form In-doped CoSb 3− s In s , substituting for Co at the 8 c sites in the irregular Sb 6 octahedron to form In-doped Co 1− r In r Sb 3 or simultaneously filling the icosahedron voids at the 2 a sites and substituting for Sb at the 24 g sites to form (In VF ) x 2/3 Co 4 Sb 12− x /3 (In Sb ) x /3 with charge-compensated compound defects [33] . The In K -edge XANES theoretical spectra of the In impurities at the 2 a , 24 g , 8 c and 2 a –24 g sites in CoSb 3 were calculated to identify which sites the In impurities occupy. The In K -edge XANES theoretical spectra (red solid lines symbolize ‘cal.’) of In-filled CoSb 3 for the In impurities (a) filling icosahedron voids at the 2 a sites, (b) substituting for Sb at the 24 g sites, (c) substituting for Co at 8 c sites and (d) simultaneously filling the icosahedron voids at the 2 a sites and substituting for Sb at the 24 g sites are compared with the experimental spectrum (circle lines symbolize ‘exp.’) of the A 0.25 sample ( Fig. 2 ). It is clear that only the In K -edge XANES theoretical spectrum for filling icosahedron voids is in good agreement with the experimental data; the other three cases have large discrepencies between the theoretical spectra and the experimental ones ( Fig. 2b–d ). Therefore, the In K -edge XANES spectra unequivocally suggest that the In impurities stably fill the Sb 12 icosahedron voids in CoSb 3 . 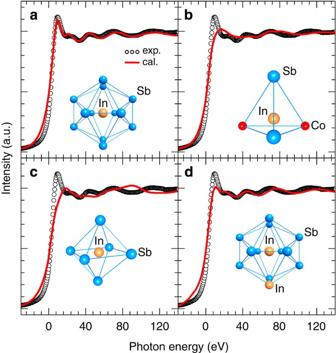Figure 2: The InK-edge XANES spectra of In impurity in CoSb3. (a) Filling Sb12icosahedron voids at the 2asites, (b) substituting for Sb at the 24gsites, (c) substituting for Co at the 8csites and (d) simultaneously filling the icosahedron voids at the 2asites and substituting for Sb at the 24gsites. The InK-edge XANES experimental spectra of A0.25are plotted for comparison. The XANES theoretical spectra are shown with red solid lines and symbolized as ‘cal.’. The XANES experimental ones are shown with black circle lines and symbolized as ‘exp.’. Figure 2: The In K -edge XANES spectra of In impurity in CoSb 3 . ( a ) Filling Sb 12 icosahedron voids at the 2 a sites, ( b ) substituting for Sb at the 24 g sites, ( c ) substituting for Co at the 8 c sites and ( d ) simultaneously filling the icosahedron voids at the 2 a sites and substituting for Sb at the 24 g sites. The In K -edge XANES experimental spectra of A 0.25 are plotted for comparison. The XANES theoretical spectra are shown with red solid lines and symbolized as ‘cal.’. The XANES experimental ones are shown with black circle lines and symbolized as ‘exp.’. Full size image 5 p -orbital hybridization between In and Sb and its effects The total DOSs of CoSb 3 and In 0.125 Co 4 Sb 12 , and partial DOS for Co, Sb and In atoms indicate that the total DOS of In-filled In 0.125 Co 4 Sb 12 near valence band maximum (VBM) and conduction band minimum (CBM) mainly stem from Co 3 d electrons and Sb 5 p electrons ( Fig. 3 ). It can be seen that there is an extra peak of the partial DOS of Co 3 d and Sb 5 p electrons near 0.31 eV for In 0.125 Co 4 Sb 12 , which exactly corresponds to the highest peak of the partial DOS of In 5 p electrons. Particularly, the DOS Sb5 p /DOS Co3 d ratio is decreased near VBM from 2.96 for CoSb 3 to 2.08 for In 0.125 Co 4 Sb 12 and increased near CBM from 0.20 for CoSb 3 to 0.22 for In 0.125 Co 4 Sb 12 . This evolution suggests that the energy of Sb 5 p electrons and Co 3 d electrons becomes closer, and the p–d orbital hybridization between Co and Sb has thus been enhanced in In 0.125 Co 4 Sb 12 . Experimentally, the XPS spectra of Co 2 p 3/2 and 2 p 1/2 core levels of In-filled CoSb 3 are gradually shifted to higher binding energies (maximum up to 0.20 eV) as the filling fraction of the In filler increased ( Fig. 4 ). The chemical shift is less than the energy resolution of XPS (about 0.47 eV) due to too low filling fraction of the In filler; however, the chemical shift can be repeated (see Supplementary Fig. 2 ) and thus may provide a plausible evidence of enhanced p–d orbital hybridization between Co and Sb. 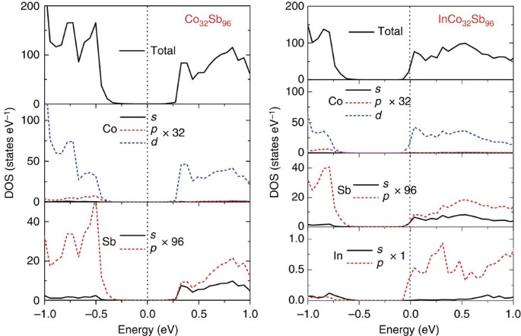Figure 3: Total DOS and partial DOS near VBM and CBM of CoSb3and In0.125Co4Sb12. The 2 × 2 × 2 supercells were calculated using projector-augmented wave method implemented in CASTEP package based on the density functional theory. Figure 3: Total DOS and partial DOS near VBM and CBM of CoSb 3 and In 0.125 Co 4 Sb 12 . The 2 × 2 × 2 supercells were calculated using projector-augmented wave method implemented in CASTEP package based on the density functional theory. 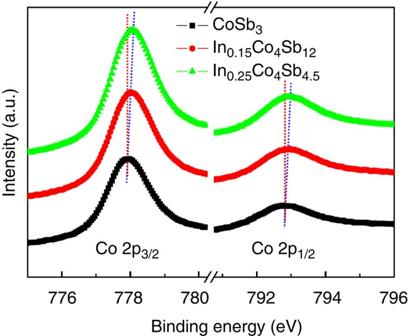Figure 4: XPS spectra of Co 2p3/2and 2p1/2core levels for CoSb3and In-filled CoSb3. Measurements were performed under the CAE mode with pass energy of 25 eV, step size of 0.05 eV and 128 scans with a Thermo VG Multilab 2000 spectrometer. Full size image Figure 4: XPS spectra of Co 2 p 3/2 and 2 p 1/2 core levels for CoSb 3 and In-filled CoSb 3 . Measurements were performed under the CAE mode with pass energy of 25 eV, step size of 0.05 eV and 128 scans with a Thermo VG Multilab 2000 spectrometer. Full size image To clarify the origin of enhanced p–d orbital hybridization between Co and Sb in In-filled CoSb 3 , the partial DOS of In atoms in the range of −12~2 eV have been analysed. We discover that the partial DOS of In 5 s electrons are distributed about 1.0 eV below the Fermi level (see Supplementary Fig. 3 ). Therefore, all In 5 s electrons are confined at the deep locations of the valence band and have no contribution to n . Although there are a few In 5 p electrons below the Fermi level, the partial DOS of In 5 p electrons are mainly distributed above and near the Fermi level, suggesting that the In 5 p electrons are almost lost in In-filled CoSb 3 . The electronic states of the In impurity clearly show that the effective charge of the In filler is smaller than, but very close to, +1. Therefore, the electronic configuration of the In filler is 5 s 2 4 d 10 5 p 0 , suggesting that the In filler may provide three unoccupied 5 p orbitals for a 5 p -orbital hybridization between In and Sb. This is corroborated by the differential charge density of In 0.125 Co 4 Sb 12 projected on the (111) plane ( Fig. 5 ) clearly showing the 5 p -orbital hybridization between In and Sb in In-filled CoSb 3 . Therefore, the enhancement in p–d orbital hybridization between Co and Sb in In-filled CoSb 3 must originate from the 5 p -orbital hybridization between In and Sb. Note that the charge density decreases between Sb and Sb atoms while it increases between In and Sb atoms for In-filled icosahedron voids, indicating that the partial charges are transferred from Sb to In, which are in good agreement with our previous XPS results [27] . Namely, the 5 p -orbital hybridization between In and Sb in In-filled CoSb 3 can still cause a charge transfer from Sb to In and produce two types of atomic-scale electric fields near the In-filled Sb 12 icosahedron, which are the atomic-scale electric fields with positive charge at the framework of In-filled Sb 12 icosahedron and the atomic-scale electric fields with negative charge in the Sb 12 icosahedron. Since the framework of Sb 12 icosahedron acts as the passage of majority carriers (electrons) in In-filled CoSb 3 , the atomic-scale electric fields with positive charge at the framework of In-filled Sb 12 icosahedron may accelerate electron movement. 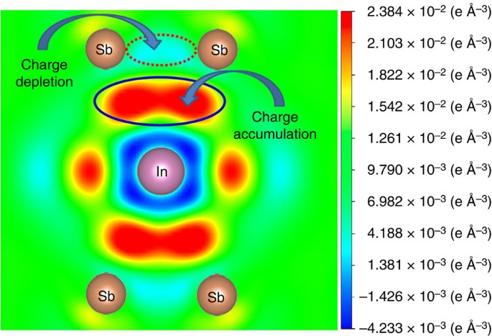Figure 5: Differential charge density of In0.125Co4Sb12projected on the (111) plane. The 2 × 2 × 2 supercells were calculated using the projector-augmented wave method implemented in CASTEP package based on the density functional theory. The differential charge density. deltap=pInCo32Sb96−pCo32Sb96−pIn Figure 5: Differential charge density of In 0.125 Co 4 Sb 12 projected on the (111) plane. The 2 × 2 × 2 supercells were calculated using the projector-augmented wave method implemented in CASTEP package based on the density functional theory. The differential charge density. delta p = p InCo32Sb96 − p Co32Sb96 − p In Full size image In–Sb weak covalent bond and its effects The extended XAFS (EXAFS) analysis reveals that the In–Sb bond length is about 3.35 Å for the A 0.2 sample (see Supplementary Fig. 4 ) and very close to the value (3.36 Å) reported for In 0.2 Co 4 Sb 12 (ref. 34 ), while it is only about 2.81 Å for InSb [43] . The longer In–Sb bond indicates less orbital overlapping and weakened repulsion interaction between bonding and antibonding states of In–Sb bond in In-filled CoSb 3 . Therefore, the In–Sb bond between In filler and host framework of Sb 12 icosahedron must be a weak covalent bond in In-filled CoSb 3 , further corroborating the lower energy of the main peak A 3 than that of A 2 ( Fig. 1 ). Obviously, the In fillers can rattle inside the voids and cause heat-carrying phonon-localized resonant scattering, thereby remarkably reducing κ L . The temperature dependences of κ L values for CoSb 3 and In-, Ba- and Ga-filled CoSb 3 ( Fig. 6 ) show that κ L value at 300 K is only about 5.16 W m −1 K −1 for In 0.08 Co 4 Sb 12 and 3.75 W m −1 K −1 for In 0.18 Co 4 Sb 12 while more than 10 W m −1 K −1 for CoSb 3 . The κ L values of In 0.08 Co 4 Sb 12 are smaller than those of Ba 0.09 Co 4 Sb 12 in the range of 300–650 K, suggesting that the In filler is more effective in reducing κ L than Ba at a comparable filling fraction. The κ L values of In 0.08 Co 4 Sb 12 , however, are significantly greater than those of Ga 0.09 Co 4 Sb 12 in the range of 300–800 K, suggesting different doping behaviour in CoSb 3 between In and Ga. The lower κ L values of Ga 0.09 Co 4 Sb 12 are due to the additional defect scattering induced by the Sb-substitutional Ga, because Ga impurties in CoSb 3 were thought to simultaneously occupy both the icosahedron voids and the Sb sites [32] . 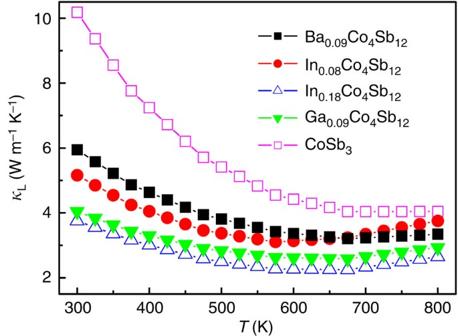Figure 6: Temperature dependences of lattice thermal conductivity in the range of 300–800 K. The data of CoSb3are plotted for comparison with those of In-, Ba-, and Ga-filled CoSb3. Figure 6: Temperature dependences of lattice thermal conductivity in the range of 300–800 K. The data of CoSb 3 are plotted for comparison with those of In-, Ba-, and Ga-filled CoSb 3 . Full size image The n values of In 0.18 Co 4 Sb 12 are almost the same as those of Ba 0.09 Co 4 Sb 12 in the range of 100–300 K ( Fig. 7 ), clearly indicating that the In filler provides one electron and is univalent (In + ) in In-filled CoSb 3 because the Ba filler provides two electrons in Ba-filled CoSb 3 . The electronic structure of the In filler described above not only is the physical mechanism of low n for In-filled CoSb 3 , but also may reasonably explain why the n values of In 0.18 Co 4 Sb 12 and Ba 0.09 Co 4 Sb 12 are very close in the range of 100–300 K. At the same time, the charge transfer from Sb to In in In-filled CoSb 3 must produce the same amount of atomic-scale electric fields with positive charge at the framework of In-filled Sb 12 icosahedron; therefore, the major carriers (electrons) nearby the In-filled Sb 12 icosahedron are not only partially annihilated but also accelerated because of the attraction by the atomic-scale electric fields with positive charge. These multi-functional local transport effects may explain that the In-filled CoSb 3 has higher μ H than those of Ba-filled and Ga-filled CoSb 3 in the range of 100–300 K under comparable n values ( Fig. 8 ). As a result, the In-filled CoSb 3 have higher σ than Ba- and Ga-filled CoSb 3 in the range of 150–800 K, although their n values are very close ( Fig. 9 ), which can be attributed to an increase in μ H induced by accelerated electron movement nearby the In-filled Sb 12 icosahedron. Compared with Ba- and In-filled CoSb 3 , the lower μ H of Ga-filled CoSb 3 in the range of 10–100 K may be reasonably explained by the dual-site occupancy of Ga impurity in CoSb 3 (ref. 32 ). In addition, the μ H values of Ba- and In-filled CoSb 3 share similar temperature dependence in the range of 10–300 K ( Fig. 8 ), implying that the electron scattering mechanisms are the same for both cases and there is thus no case of In occupying at the Sb sites. This is well consistent with the XANES results as shown in Fig. 2 . 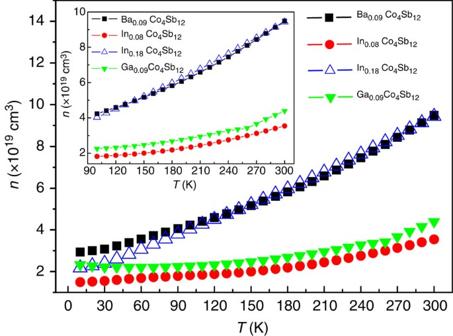Figure 7: Temperature dependences of carrier concentration in the range of 10–300 K. The inset shows the temperature dependences of carrier concentration of In-, Ba-, and Ga-filled CoSb3in the range of 100–300K. Figure 7: Temperature dependences of carrier concentration in the range of 10–300 K. The inset shows the temperature dependences of carrier concentration of In-, Ba-, and Ga-filled CoSb 3 in the range of 100–300K. 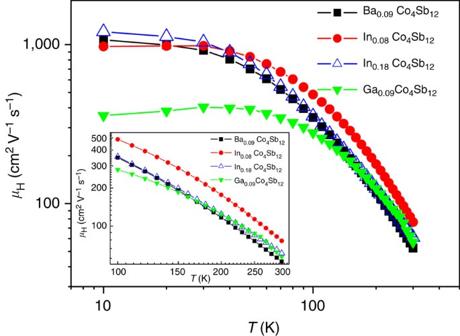Figure 8: Temperature dependences of Hall mobility in the range of 10–300 K. The inset shows the temperature dependences of Hall mobility of In-, Ba-, and Ga-filled CoSb3in the range of 100–300K. Full size image Figure 8: Temperature dependences of Hall mobility in the range of 10–300 K. The inset shows the temperature dependences of Hall mobility of In-, Ba-, and Ga-filled CoSb 3 in the range of 100–300K. 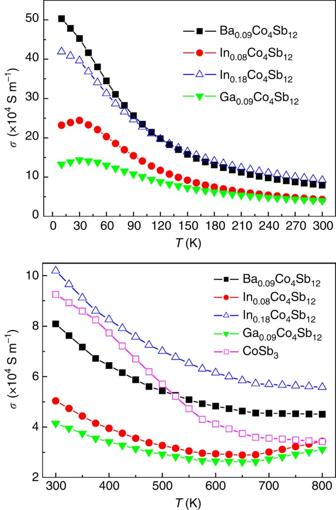Figure 9: Temperature dependences of electrical conductivity in the range of 10–800 K. The data of CoSb3in the range of 300–800K are plotted for comparison with those of In-, Ba-, and Ga-filled CoSb3. Full size image Figure 9: Temperature dependences of electrical conductivity in the range of 10–800 K. The data of CoSb 3 in the range of 300–800K are plotted for comparison with those of In-, Ba-, and Ga-filled CoSb 3 . Full size image The enhancement of the p–d orbital hybridization between Co and Sb induced by the In filler still provides a more reasonable explanation for the band structure of In 0.125 Co 4 Sb 12 . Compared with CoSb 3 (see Supplementary Fig. 5 ), the Fermi level of In 0.125 Co 4 Sb 12 is migrated into conduction bands and the energy gap between the Fermi level and CBM at H , N and P points with high symmetry is significantly decreased from 0.45~0.35 eV for CoSb 3 to 0.12~0.03 eV for In 0.125 Co 4 Sb 12 . As a result, the DOS of VBM is significantly decreased while the DOS of CBM is remarkably increased. Namely, there is an asymmetric distribution of DOS near the Fermi level of In-filled CoSb 3 beneficial to obtaining a large α . Such a DOS asymmetric distribution may very well explain why the absolute α values of In-filled CoSb 3 are higher than those of n -type Ba-, Sr-, Yb- and Nd-filled CoSb 3 , with similar n on the order of 10 19 cm −3 at room temperature [25] , [44] , [45] , [46] , [48] , [49] , as shown in Fig. 10 . The α values at 300 K reached 259 μV K −1 for In 0.08 Co 4 Sb 12 with 3.5 × 10 19 cm −3 and 198 μV K −1 for In 0.18 Co 4 Sb 12 with 9.4 × 10 19 cm −3 . Obviously, the large α values of In-filled CoSb 3 originate from the increase in DOS of CBM near the Fermi level due to enhanced p–d orbital hybridization between Co and Sb induced by the In filler. 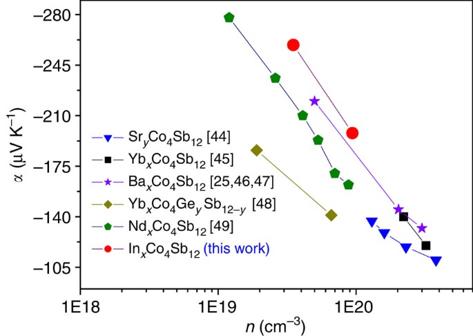Figure 10: Carrier concentration dependences of the Seebeck coefficient ofn-type filled CoSb3at room temperature. Here, compare the data of Sr-, Yb-, Ba-, Nd-, and In-filled CoSb3with n on the order of 1019~1020cm−3. Figure 10: Carrier concentration dependences of the Seebeck coefficient of n -type filled CoSb 3 at room temperature. Here, compare the data of Sr-, Yb-, Ba-, Nd-, and In-filled CoSb 3 with n on the order of 10 19 ~10 20 cm −3 . Full size image Therefore, the perfect combination of low κ L , high σ and large α for In-filled CoSb 3 originates from the following physical and chemical mechanisms. First, the low κ L is due to the heat-carrying phonon-localized resonant scattering induced by In-filler rattling. Second, the high σ is attributed to the accelerated electron movement induced by the charge transfer from Sb to In. Third, the large α benefits from the increase in DOS of CBM near the Fermi level induced by the enhanced p–d orbital hybridization between Co and Sb. The 5 p -orbital hybridization between In and Sb in In-filled CoSb 3 can cause a charge transfer from Sb to In and the enhancement of p–d orbital hybridization between Co and Sb. The fundamental origin of low n of In-filled CoSb 3 is that all 5 s electrons of the In filler are confined at the deep locations of the valence band. The low n and asymmetric distribution of DOS near the Fermi level provide a favourable condition for adjusting σ and α of In-filled CoSb 3 in an independent way. Synthesis and characterization In-filled In x Co 4 Sb 12 ( x =0.1, 0.2 and 0.25) bulk materials were prepared by a combination of melting, annealing and spark plasma sintering reported elsewhere [25] . Another three bulk materials (CoSb 3 , Ba 0.1 Co 4 Sb 12 and Ga 0.1 Co 4 Sb 12 ) were prepared with the same method for comparsion. X-ray diffraction (PANalytical X’ Pert PRO) and scanning electron microscope analysis confirmed that all the annealed samples In x Co 4 Sb 12 ( x =0.1, 0.2 and 0.25) were composed of single-phase skutterudite, while all the quenched samples consisted of Sb, CoSb, CoSb 2 and InSb. Chemical compositions of all the bulk materials were determined by electron probe microanalysis (EPMA, JXA-8230). XANES and EXAFS of quenched In 0.2 Co 4 Sb 12 and annealed In x Co 4 Sb 12 samples were measured under a working voltage of 3.5 GeV and a working current of 300 mA at BL14W1 beamline in the Shanghai Synchrotron Radiation Facility (SSRF). A Si (311) double-crystal monochromater with energy resolution of 0.5 × 10 −4 eV@10 keV was employed to measure In K -edge spectra. All XANES and EXAFS spectra were measured three times to ensure reproducibility. The In K -edge XANES spectra of InSb and the In metal were also recorded for comparison. XPS of Co 2 p 3/2 and 2 p 1/2 core levels were recorded at pass energy of of 25 eV, step size of 0.05 eV and 128 scans with Thermo VG Multilab 2000 spectrometer. Transport measurement The σ and α values were measured with the standard four-probe method (UlvacRiko: ZEM-3) in Ar atmosphere. The κ was calculated using the equation κ=DρC p , where C p is the specific heat capacity, ρ the bulk density and D the thermal diffusion coefficient. D was measured by a laser flash technique (Netzsch LFA 427) in a flowing Ar atmosphere, C p with a TA Q20 differential scanning calorimeter and ρ by Archimedes method. κ L was obtained by subtracting the electrical contribution from κ using the equation κ L = κ − κ E . κ E is expressed by the Wiedemann–Franz κ E = σLT , where L is the Lorenz number. Uncertainties are ±5–7% for σ and κ L , and ±5% for α . The n and μ H were measured under 10–300 K with Quantum Design PPMS. Theoretical calculation The K -edge XANES theoretical spectra of In impurity at four kinds of crystallographic sites (2 a , 24 g , 8 c and 2 a –24 g ) in CoSb 3 were calculated with the self-consistent multiple-scattering theory based on real-space clusters implemented in FEFF9 package [50] . The In K -edge EXAFS experimental spectra were first normalized and background subtracted to obtain the k -weighted spectra, and then Fourier transformed to obtain the length of the In–Sb bond. The DOSs, band structure and differential charge densities projected on the (111) plane of CoSb 3 and In 0.125 Co 4 Sb 12 using a 2 × 2 × 2 supercell were calculated using a projector-augmented wave method implemented in CASTEP package based on the density functional theory [51] . Lattice relaxation and structural optimization were carried out through total energy calculations. How to cite this article: Zhao, W. et al . Multi-localization transport behaviour in bulk thermoelectric materials. Nat. Commun. 6:6197 doi: 10.1038/ncomms7197 (2015).